Dependence of fertility on kisspeptin–Gpr54 signaling at the GnRH neuron Signaling between kisspeptin and its receptor, G-protein-coupled receptor 54 (Gpr54), is now recognized as being essential for normal fertility. However, the key cellular location of kisspeptin–Gpr54 signaling is unknown. Here we create a mouse with a GnRH neuron-specific deletion of Gpr54 to assess the role of gonadotropin-releasing hormone (GnRH) neurons. Mutant mice are infertile, fail to go through puberty and exhibit markedly reduced gonadal size and follicle-stimulating hormone levels alongside GnRH neurons that are unresponsive to kisspeptin. In an attempt to rescue the infertile phenotype of global Gpr54 −/− mutants, we use BAC transgenesis to target Gpr54 to the GnRH neurons. This results in mice with normal puberty onset, estrous cyclicity, fecundity and a recovery of kisspeptin’s stimulatory action upon GnRH neurons. Using complimentary cell-specific knockout and knockin approaches we demonstrate here that the GnRH neuron is the key site of kisspeptin–Gpr54 signaling for fertility. The importance of kisspeptin and G-protein-coupled receptor 54 (GPR54) (also known as KISS1R) to fertility was signalled by the seminal discovery in 2003 of human pedigrees with GPR54 mutations that failed to go through puberty [1] , [2] . Large numbers of clinical and laboratory studies have since shown that kisspeptin–Gpr54 signaling is essential for normal fertility in all mammalian species [3] , [4] , [5] , [6] , [7] . However, kisspeptin and Gpr54 are expressed throughout the body, including the pituitary gland, gonads and placenta where they have been proposed to have several important roles in reproduction [8] , [9] , [10] , [11] , [12] , [13] . Furthermore, kisspeptin has been shown to exert its effects on the activity of multiple different hypothalamic cell populations [14] , [15] , [16] . At present, the relative importance of kisspeptin–Gpr54 signaling to fertility at different sites within the hypothalamo–pituitary–gonadal (HPG) axis is unknown. The gonadotropin-releasing hormone (GnRH) neurons in mammals express Gpr54 (refs 17 , 18 , 19 ), and kisspeptin has potent effects on GnRH neuron excitability [20] , [21] , [22] , [23] , [24] , demonstrating that this is a locus for kisspeptin’s actions within the HPG axis. To establish the importance of kisspeptin–Gpr54 signaling at the GnRH neuron for fertility, two genetic approaches were undertaken. In the first, we generated a mouse in which Gpr54 was floxed and crossed with an established GnRH-Cre line to generate mutant mice carrying a GnRH neuron-targeted deletion of Gpr54 . In the second, we set out to rescue the infertile phenotype of the Gpr54 null mouse by re-introducing functional Gpr54 selectively to the GnRH neurons. Both approaches reveal that the critical site of kisspeptin action to regulate fertility in the mouse is at the GnRH neuron. Generation of GnRH neuron-specific Gpr54-deleted mice Gpr54 loxP/loxP (Gpr54 f/f ) mice were generated by gene targeting in mouse embryonic stem cells (ES). Positive ES clones were used to produce animals with LoxP sites flanking exon two of Gpr54 ( Fig. 1a ). The Gpr54 f/f mice were crossed with a GnRH-Cre line [25] to generate mice in which Gpr54 was deleted from the GnRH neurons (GnRH-Cre +/− ;Gpr54 f/f ). The well-characterized GnRH-Cre line targets essentially all GnRH neurons [25] , [26] . To characterize these mice further, we crossed female GnRH-Cre mice with a ROSA26::LoxP-Stop-LoxP-LacZ reporter line [27] and found that 98±1% (s.e.m.) of GnRH neurons expressed Xgal in the form of small blue intracytoplasmic dots, typical for this phenotype [28] ( n =6; Fig. 1b ). We also detected Xgal-expressing cells in the intermediate division of the lateral septum (LSi) and bed nucleus of the stria terminalis (BNST). These represent sites where GnRH is expressed transiently in the early postnatal period in the mouse brain [28] . 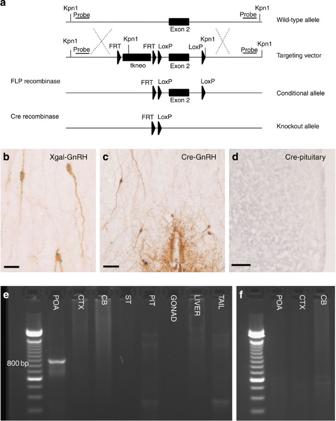Figure 1: Generation and characterization of GnRH-Cre;Gpr54 mice. (a) Schematic diagram showing the strategy for floxing exon 2 ofGpr54. (b) Dual-label for Xgal (blue cytoplasmic dots) and GnRH (brown cytoplasm) showing three GnRH neurons expressing Xgal in a GnRH-Cre;ROSA26::loxP-Stop-LoxP-LacZ27mouse cross. (c) Dual-label for Cre (black nuclei) and GnRH (brown cytoplasm) in the rostral preoptic area of GnRH-Cre mice showing the selective expression of Cre in the GnRH neurons. (d) There is a complete absence of Cre immunoreactivity in the pituitary gland. (e) Gel showing 836 bp PCR product representing recombinedGpr54allele in the preoptic area (POA) but not the neocortex (CTX), cerebellum (CB), striatum (ST), pituitary gland (PIT), ovary (GONAD), liver and tail of a female GnRH-Cre;Gpr54f/fmouse. (f) Gpr54f/f;GnRH-Cre –ve mice exhibited no 800-bp bands in the POA or elsewhere (only CTX and CB shown). Scale bars in (b) represent 20 μm,c,d=50 μm. Figure 1: Generation and characterization of GnRH-Cre;Gpr54 mice. ( a ) Schematic diagram showing the strategy for floxing exon 2 of Gpr54 . ( b ) Dual-label for Xgal (blue cytoplasmic dots) and GnRH (brown cytoplasm) showing three GnRH neurons expressing Xgal in a GnRH-Cre; ROSA26::loxP-Stop-LoxP-LacZ [27] mouse cross. ( c ) Dual-label for Cre (black nuclei) and GnRH (brown cytoplasm) in the rostral preoptic area of GnRH-Cre mice showing the selective expression of Cre in the GnRH neurons. ( d ) There is a complete absence of Cre immunoreactivity in the pituitary gland. ( e ) Gel showing 836 bp PCR product representing recombined Gpr54 allele in the preoptic area (POA) but not the neocortex (CTX), cerebellum (CB), striatum (ST), pituitary gland (PIT), ovary (GONAD), liver and tail of a female GnRH-Cre;Gpr54 f/f mouse. ( f ) Gpr54 f/f ;GnRH-Cre –ve mice exhibited no 800-bp bands in the POA or elsewhere (only CTX and CB shown). Scale bars in ( b ) represent 20 μm, c , d =50 μm. Full size image We further assessed the degree to which Gpr54 might be altered outside the brain in GnRH-Cre +/− ;Gpr54 f/f mice by examining for the presence of Cre in peripheral tissues and determining organs in which Cre-LoxP recombination occurred. Immunohistochemistry in adult female GnRH-Cre mice revealed the presence of nuclear-located Cre in GnRH neurons within the brain ( Figs1c and 2a ) but not elsewhere in the HPG axis including the pituitary ( Fig. 1d ), ovaries or testes ( n =4; Fig. 2a ). PCR using a primer set that detects Cre-recombined Gpr54 was conducted in the preoptic area (location of the GnRH neurons), neocortex, cerebellum, striatum, pituitary gland, ovary, liver and tail of female mutant GnRH-Cre +/− ;Gpr54 f/f and littermate control Gpr54 f/f mice ( n =2, each). This showed that Gpr54 was only recombined in the preoptic area and not in other tissues of GnRH-Cre +/− ;Gpr54 f/f mice ( Fig. 1e ), or anywhere in littermate Gpr54 f/f GnRH-Cre-negative mice ( Fig. 1f ). 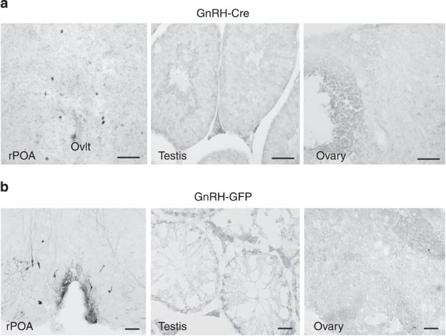Figure 2: Transgene expression in reproductive organs of GnRH-Cre and GnRH-GFP transgenic mice. (a) Immunohistochemical Ni-DAB labelling for Cre in transgenic GnRH-Cre mice showing the region of the GnRH neuron cell bodies in the rostral preoptic area (rPOA), testis and ovary. Note that Cre-immunoreactive nuclei are identified in the rPOA but not in other tissues. These Cre-positive nuclei belong to GnRH neurons (seeFig. 1c). Scale bar=20 μm. (b) Immunohistochemical Ni-DAB labelling for GFP in transgenic GnRH-GFP mice. Note that GFP-positive cell bodies and fibres are detected in the rPOA (representing GnRH neurons) but not in the testis or ovary. Scale bar=20 μm. Figure 2: Transgene expression in reproductive organs of GnRH-Cre and GnRH-GFP transgenic mice. ( a ) Immunohistochemical Ni-DAB labelling for Cre in transgenic GnRH-Cre mice showing the region of the GnRH neuron cell bodies in the rostral preoptic area (rPOA), testis and ovary. Note that Cre-immunoreactive nuclei are identified in the rPOA but not in other tissues. These Cre-positive nuclei belong to GnRH neurons (see Fig. 1c ). Scale bar=20 μm. ( b ) Immunohistochemical Ni-DAB labelling for GFP in transgenic GnRH-GFP mice. Note that GFP-positive cell bodies and fibres are detected in the rPOA (representing GnRH neurons) but not in the testis or ovary. Scale bar=20 μm. Full size image Together, these characterization studies demonstrate that Cre is directed to all (98%) GnRH neurons as well as, developmentally, to scattered cells in the LSi and BNST in the brain, but not to other tissues. Whereas no cells in the BNST express endogenous Gpr54, a very few can be found in the LSi [18] . As a result, Gpr54 will be deleted from essentially all GnRH neurons and, possibly, from a very small population of LSi cells in GnRH-Cre +/− ;Gpr54 f/f mice. To check whether Gpr54 was in fact deleted from the GnRH neurons in this mutant mouse line, GnRH-Cre +/− ;Gpr54 f/f mice were crossed to a GnRH-green fluorescent protein (GFP)-transgenic line [29] to enable electrophysiological recordings of the GnRH neurons in the acute brain-slice preparation. Previous studies have shown that kisspeptin acts directly on ~75% of the GnRH neurons to generate potent excitatory actions in this preparation [20] , [21] , [22] , [23] , [24] . Cell-attached recordings of the GnRH neurons were undertaken in the absence or presence of an amino-acid receptor blocker (AAB) cocktail that reduces the likelihood of recording any indirect effects of kisspeptin on the GnRH neurons. Adult female (age 69±2 (s.e.m.) days) littermate control (GnRH-GFP +/− ;GnRH-Cre +/− ;Gpr54 flox-htz) and mutant (GnRH-GFP +/− ;GnRH-Cre +/− ;Gpr54 f/f ) mice were used. In control littermate mice, 9 of 14 GnRH neurons from 3 mice responded to the 100-nM kisspeptin with the typical prolonged pattern of increased firing both in the absence and presence of the AAB cocktail ( Fig. 3a ). In mutants, 19 GnRH neurons were examined from four mice, with none being excited by the 100-nM kisspeptin, again regardless of whether the AAB cocktail was used ( Fig. 3b ). The basal firing rate of the GnRH neurons was different between the two groups, being 0.84±0.7 Hz in controls and 0.16±0.02 Hz (s.e.m.) in mutants ( P <0.01; analysis of variance (ANOVA), post hoc Tukey test). The AAB cocktail itself had no significant effects on basal firing in either genotype ( P >0.05; paired sample Wilcoxon rank test). These data demonstrate that Gpr54 signaling has been deleted completely at the GnRH neuron in GnRH-Cre +/− ;Gpr54 f/f mice. 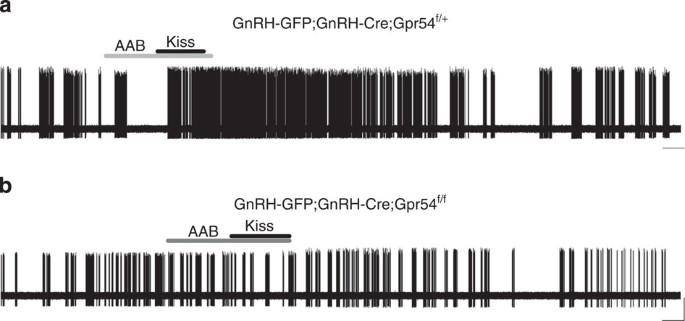Figure 3: Absence of kisspeptin activation of GnRH neurons in GnRH-Cre+/−;Gpr54f/fmice. (a) Cell-attached recording from a GnRH neuron in a control GnRH-GFP mouse showing the normal strong activation by the 100-nM kisspeptin (Kiss). The cell was first treated with an AAB cocktail to block any indirect actions of kisspeptin through glutamate or GABAAionotropic receptors. (b) The activation of GnRH neurons by kisspeptin is lost in GnRH neurons from GnRH-Cre+/−;Gpr54f/fmice. Scale bars represent 1 min (horizontal) and 1 mV (vertical). Figure 3: Absence of kisspeptin activation of GnRH neurons in GnRH-Cre +/− ;Gpr54 f/f mice. ( a ) Cell-attached recording from a GnRH neuron in a control GnRH-GFP mouse showing the normal strong activation by the 100-nM kisspeptin (Kiss). The cell was first treated with an AAB cocktail to block any indirect actions of kisspeptin through glutamate or GABA A ionotropic receptors. ( b ) The activation of GnRH neurons by kisspeptin is lost in GnRH neurons from GnRH-Cre +/− ;Gpr54 f/f mice. Scale bars represent 1 min (horizontal) and 1 mV (vertical). Full size image Phenotype of GnRH neuron-specific Gpr54-deleted mice GnRH neuron-selective deletion of Gpr54 resulted in mice that appeared normal in all respects other than a failure to go through puberty, reduced gonadal size and subsequent infertility. GnRH-Cre +/− ;Gpr54 f/f mutants failed to exhibit vaginal opening (assessed up to 6 months age) and, as with male mutants, were infertile ( n =12 per sex). Compared with control littermate Gpr54 f/f mice, GnRH-Cre +/− ;Gpr54 f/f mutants exhibited testis and ovarian tissue weights that were reduced by over 90% in both sexes (testis: control 91±22 mg (s.e.m. ), mutant 4.5±1.4 mg ( n =7 each, P <0.01, Mann–Whitney U -test, Fig. 4b ); ovary: control 18.0±0.3 mg, mutant 3.0±0.1 mg ( n =10 each, P <0.01, Mann–Whitney U -test) ( Fig. 4a ). Histological examination revealed the absence of sperm in testes ( Fig. 5a,b ) and corpora lutea in the ovary ( Fig. 5c,d ). The distribution and numbers of the GnRH neurons were not altered in GnRH-Cre +/− ;Gpr54 f/f mice. Mice carrying the GnRH-Cre transgene but heterozygous for the floxed Gpr54 were normal in all respects including their fertility. 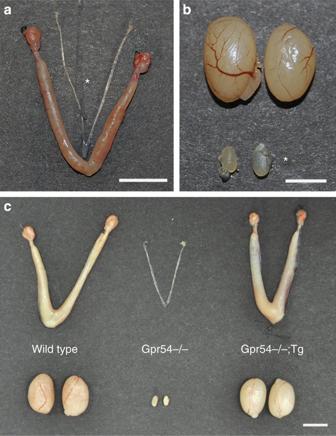Figure 4: Gonads of GnRH neuron Gpr54-related mutant mice. (a) Uteri and ovaries and (b) testes of a wild-type and GnRH-Cre+/−;Gpr54f/fmice (indicated by *). (c) Uteri, ovaries and testes of wild-type, Gpr54−/−and Gpr54−/−;Tg rescue mice. Scale bars=5 mm. Figure 4: Gonads of GnRH neuron Gpr54-related mutant mice. ( a ) Uteri and ovaries and ( b ) testes of a wild-type and GnRH-Cre +/− ;Gpr54 f/f mice (indicated by *). ( c ) Uteri, ovaries and testes of wild-type, Gpr54 −/− and Gpr54 −/− ;Tg rescue mice. Scale bars=5 mm. 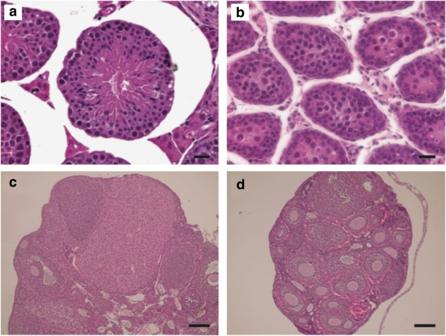Figure 5: Gonadal histology of GnRH-Cre;Gpr54f/fand littermate control Gpr54f/fmice. (a,b) Testis morphology in adult Gpr54f/f(a) and GnRH-Cre+/−; Gpr54f/f(b) mice. No spermatozoa are observed in the seminiferous tubules of the GnRH-Cre+/−; Gpr54f/fmice (b) as compared with the Gpr54f/flittermates; scale bars ina,brepresent 100 μm (n=4–6 per group). (c,d) Ovarian morphology in adult Gpr54f/f(c) and GnRH-Cre+/−; Gpr54f/f(d) mice. Whereas corpora lutea were readily observed in the ovaries of Gpr54f/fmice (c), none were observed in the ovaries of GnRH-Cre+/−; Gpr54f/fmice (d); scale bars inc,drepresent 1 mm (n=5 per group). Full size image Figure 5: Gonadal histology of GnRH-Cre;Gpr54 f/f and littermate control Gpr54 f/f mice. ( a , b ) Testis morphology in adult Gpr54 f/f ( a ) and GnRH-Cre +/− ; Gpr54 f/f ( b ) mice. No spermatozoa are observed in the seminiferous tubules of the GnRH-Cre +/− ; Gpr54 f/f mice ( b ) as compared with the Gpr54 f/f littermates; scale bars in a , b represent 100 μm ( n =4–6 per group). ( c , d ) Ovarian morphology in adult Gpr54 f/f ( c ) and GnRH-Cre +/− ; Gpr54 f/f ( d ) mice. Whereas corpora lutea were readily observed in the ovaries of Gpr54 f/f mice ( c ), none were observed in the ovaries of GnRH-Cre +/− ; Gpr54 f/f mice ( d ); scale bars in c , d represent 1 mm ( n =5 per group). Full size image Basal luteinizing hormone (LH) levels in adult male littermate controls (Gpr54 f/f ) and mutants (GnRH-Cre +/− ;Gpr54 f/f ) were, respectively, 0.65±0.34 (s.e.m.) ( n =6) versus 0.13±0.03 ng ml −1 ( n =6) ( P >0.05; Mann–Whitney U -test), while follicle-stimulating hormone (FSH) concentrations were 13.4±1.04 versus 0.25±0.01 ng ml −1 ( P <0.01; Mann–Whitney U -test). To provide an in vivo functional assay of the ability of the GnRH neuronal network to respond to kisspeptin, adult male mice ( n =5) were given 100 nmol kisspeptin i.p. This evoked a significant sevenfold (4.5±0.4 ng ml −1 (s.e.m. ); P <0.05, Mann–Whitney U -test) increase in LH secretion 10 min later in littermate control mice but had no effect in mutant mice (post kisspeptin=0.2±0.1 ng ml −1 ; n =4). These observations demonstrate that GnRH-Cre +/− ;Gpr54 f/f mice are infertile, fail to go through puberty, are unresponsive to kisspeptin and exhibit markedly reduced gonadal size and reduced circulating FSH levels. Generation of GnRH neuron-specific Gpr54 rescue mice The above experiments indicated that Gpr54 signaling at the GnRH neuron was essential for fertility. As such, we hypothesized that the selective re-introduction of Gpr54 to GnRH neurons in infertile global Gpr54 −/− mice might rescue their fertility. To do this, we used BAC transgenesis to generate rescue mice (Gpr54 −/− ;Tg) that express Gpr54 under the control of GnRH gene-regulatory elements on a Gpr54 −/− mutant background [30] ( Fig. 6a ). The ability of this strategy to target GnRH neuron selectively was assessed by generating other mouse lines at the same time with the same ~200-kb BAC but coding for GFP (GnRH-GFP). Four lines of GnRH-GFP mice were generated, each of which had exactly the same expression phenotype with the transgene targeted to >95% of GnRH neurons ( Fig. 6b ), as well as a population of cells residing in the LSi but not in the pituitary gland, ovary or testis ( Fig. 2b ). This indicates that the GnRH BAC used in these studies accurately targets transgene expression to GnRH neurons and LSi cells. 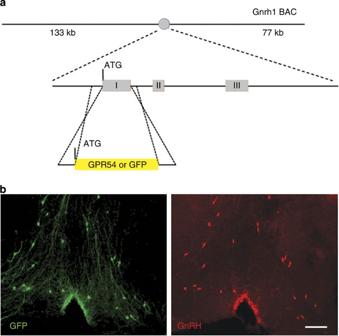Figure 6: Generation of Gpr54−/−-Tg rescue mice and selective targeting of transgene to GnRH neurons. (a) Schematic of the GnRH-BAC transgene harboring either GPR54 or GFP. (b) Dual immunofluorescence showing the expression of GFP (green) and GnRH (red) in the rostral preoptic area of a GnRH-BAC-GFP mouse. Note the complete overlap between GnRH cell body immunofluorescence and GFP expression. Scale bar =100 μm. Figure 6: Generation of Gpr54 −/− -Tg rescue mice and selective targeting of transgene to GnRH neurons. ( a ) Schematic of the GnRH-BAC transgene harboring either GPR54 or GFP. ( b ) Dual immunofluorescence showing the expression of GFP (green) and GnRH (red) in the rostral preoptic area of a GnRH-BAC-GFP mouse. Note the complete overlap between GnRH cell body immunofluorescence and GFP expression. Scale bar =100 μm. Full size image As the Gpr54 −/− mouse line used in the rescue studies is a translational knockout, it was not useful to evaluate Gpr54 transcript expression in these studies. As such, to check that the transgene did not target cells outside the GnRH/LSi, we established a functional in vitro assay of kisspeptin action in the pituitary gland, a tissue within the HPG axis where kisspeptin–Gpr54 signaling is documented [11] . As Gpr54 receptor signaling modulates both ERK1/2 and Akt phosphorylation status [31] , we examined the ability of the 10-nM kisspeptin to modulate ERK1/2 and Akt phosphorylation using western blot (full membranes in Supplementary Fig. S1 ) in littermate adult female Gpr54 −/− and Gpr54 −/− ;Tg mutants and wild-type mice ( n =8 each; Fig. 7 ). To normalize circulating estradiol levels between the three gentoypes, all mice were given estradiol implants for 2 weeks prior to experimentation. Whereas kisspeptin treatment significantly reduced levels of phosphorylated ERK1/2 ( P <0.01, Mann–Whitney U -test) and Akt ( P <0.01) by >25% in wild-type mice, it had no effect ( P >0.05) in global Gpr54 −/− mice or in rescue Gpr54 −/− ;Tg animals ( Fig. 7 ). This demonstrates that the GnRH neuron-targeting strategy does not rescue kisspeptin signaling in the pituitary gland. 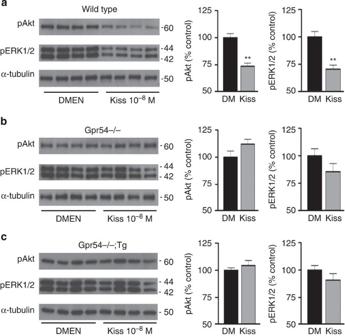Figure 7: Suppression of Akt and ERK1/2 phosphorylation by kisspeptin in the pituitary gland is not rescued in Gpr54−/−-Tg mice. (a) Western blot membrane showing phosphorylated Akt (pAkt), phosphorylated ERK1/2 (pERK1/2) and α-tubulin protein levels from four vehicle DMEM (DM)- and four kisspeptin-treated pituitary glands from female wild-type mice. The positions of kDa marker weights are shown to the right. Histograms to the right show mean+s.e.m. (n=4 each group) quantitated levels as a percentage of control values. Kisspeptin (10 nM) causes a significant reduction in both pAkt and pERK1/2 in wild-type mice. **P<0.01 Mann–WhitneyU-test. (b) The same experiment in global Gpr54−/−mice reveals an absence of kisspeptin action. (c) Similarly, the pituitary glands of rescue Gpr54−/−;Tg mice do not show any response to kisspeptin. Full-length immunoblots are shown inSupplementary Fig. S1. Figure 7: Suppression of Akt and ERK1/2 phosphorylation by kisspeptin in the pituitary gland is not rescued in Gpr54 −/− -Tg mice. ( a ) Western blot membrane showing phosphorylated Akt (pAkt), phosphorylated ERK1/2 (pERK1/2) and α-tubulin protein levels from four vehicle DMEM (DM)- and four kisspeptin-treated pituitary glands from female wild-type mice. The positions of kDa marker weights are shown to the right. Histograms to the right show mean+s.e.m. ( n =4 each group) quantitated levels as a percentage of control values. Kisspeptin (10 nM) causes a significant reduction in both pAkt and pERK1/2 in wild-type mice. ** P <0.01 Mann–Whitney U -test. ( b ) The same experiment in global Gpr54 −/− mice reveals an absence of kisspeptin action. ( c ) Similarly, the pituitary glands of rescue Gpr54 −/− ;Tg mice do not show any response to kisspeptin. Full-length immunoblots are shown in Supplementary Fig. S1 . Full size image To ensure that the transgene strategy had actually re-introduced functional Gpr54 to the GnRH neuronal phenotype, we crossed Gpr54 −/− ;Tg mice with the GnRH-GFP line to undertake an electrophysiological analysis of kisspeptin actions on GnRH neurons in the three genotypes. As for the GnRH neuron-selective Gpr54-deletion studies above, we undertook cell-attached recordings in the absence and presence of the AAB cocktail. In control adult female GnRH-GFP mice, the 100-nM kisspeptin was found to exert its typical, long-lasting activation of firing in 12 of the 14 (85%) GnRH neurons from six mice, regardless of the presence of the AAB cocktail ( Fig. 8a ). As expected, kisspeptin exerted no effects on 15 GnRH neurons from three global Gpr54 −/− mice ( Fig. 8b ). However, in rescue Gpr54 −/− ;Tg mice, 13 of 19 (68%) GnRH neurons from five mice exhibited the typical prolonged activation of firing in response to kisspeptin and, again, this occurred in the presence ( n =5; Fig. 8c ) and absence ( n =8) of the AAB cocktail. Significant differences existed between basal GnRH neuron-firing rates exhibited by each genotype ( Fig. 8 ); control GnRH-GFP; 0.83±0.07 Hz (s.e.m. ); global Gpr54 −/− , 0.07±0.01; Gpr54 −/− ; Tg, 5.8±0.07 Hz; P <0.01 between each group, ANOVA with post hoc Tukey tests). Treatment with the AAB cocktail had no effect ( P >0.05; paired sample Wilcoxon rank test) on the high basal firing rate of GnRH neurons in Gpr54 −/− ;Tg mice ( Fig. 8c ). These observations show that functional Gpr54 signaling has been re-introduced to the GnRH neuron in Gpr54 −/− ;Tg mice. 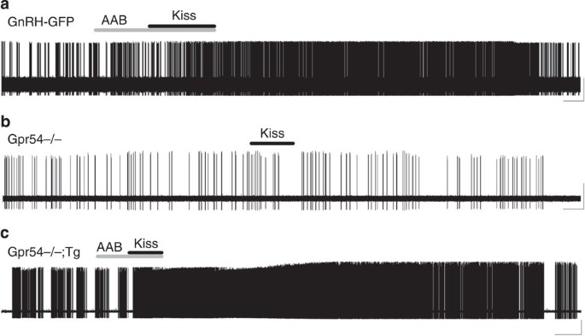Figure 8: Kisspeptin activation of GnRH neurons is rescued in Gpr54−/−-Tg mice. (a) Cell-attached recording from a GnRH neuron in a GnRH-GFP mouse showing the normal 100-nM kisspeptin (Kiss) activation of GnRH neuron firing. The cell was first treated with an AAB cocktail to block any indirect actions of kisspeptin through glutamate or GABAAionotropic receptors. (b) Kisspeptin is unable to activate GnRH neurons from Gpr54−/−mice. (c) The kisspeptin activation of GnRH neuron is recovered in rescue Gpr54−/−;Tg mice that also exhibit higher basal firing. Time scale bar (horizontal) =2 min. Vertical scale bar =0.5 mV (a) and 2 mV (b,c). Figure 8: Kisspeptin activation of GnRH neurons is rescued in Gpr54 −/− -Tg mice. ( a ) Cell-attached recording from a GnRH neuron in a GnRH-GFP mouse showing the normal 100-nM kisspeptin (Kiss) activation of GnRH neuron firing. The cell was first treated with an AAB cocktail to block any indirect actions of kisspeptin through glutamate or GABA A ionotropic receptors. ( b ) Kisspeptin is unable to activate GnRH neurons from Gpr54 −/− mice. ( c ) The kisspeptin activation of GnRH neuron is recovered in rescue Gpr54 −/− ;Tg mice that also exhibit higher basal firing. Time scale bar (horizontal) =2 min. Vertical scale bar =0.5 mV ( a ) and 2 mV ( b , c ). Full size image Phenotype of GnRH neuron-specific Gpr54 rescue mice The fertility of Gpr54 −/− mice was rescued by the transgene, with all five lines of Gpr54 −/− ;Tg mice exhibiting the same phenotype. Whereas male Gpr54 −/− mice were infertile with small testes (36±6 mg (s.e.m. )), wild-type (120±10 mg) and Gpr54 −/− ;Tg (106±12 mg) mice exhibited normal testis weights ( Fig. 4c ) and fertility ( n =5–10, Fig. 9d–f ). Wild-type and Gpr54 −/− ;Tg male mice became sexually mature at 46±1 (s.e.m.) versus 47±1 days ( n =6, each group), respectively, whereas Gpr54 −/− mice did not produce any litters ( n =9; Fig. 9d ). Subsequent mating of these mice for 4 months showed that the numbers of litters (4.9±0.4 (s.e.m.) versus 4.0±3.4; Fig. 9f ) and pups per litter ( Fig. 9e ) were the same for wild-type ( n =6) and rescue ( n =6) male mice, whereas Gpr54 −/− mice ( n =9) were infertile ( Fig. 9f ). 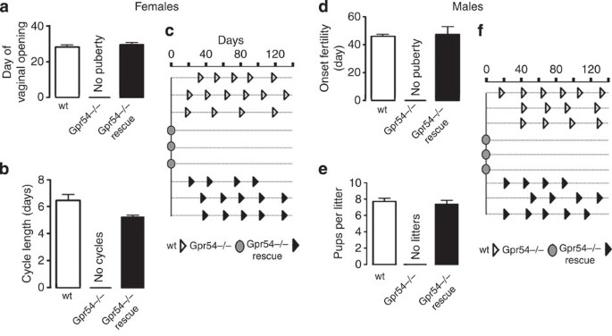Figure 9: Rescue of puberty onset and fecundity in Gpr54>−/−-Tg rescue mice. Mean+s.e.m. values showing (a) the day of vaginal opening in three genotypes (n=6 each). (b) Estrous cycle length in three genotypes (n=6 each); wild-type and Gpr54−/−;Tg rescue are not significantly different. (c) Fecundity over 120 days for three representative individual female mice (each line) from each genotype with symbols showing the times at which each litter was born. Gpr54−/−mice failed to generate any litters. (d) Onset of reproductive competence for male mice of three genotypes (n=6 each). Gpr54−/−mice failed to sire any litters. (e) Pups per litter were not different between wild-type and Gpr54−/−;Tg rescue male mice. (f) Fecundity over 120 days for three representative individual male mice (each line) from each genotype. Figure 9: Rescue of puberty onset and fecundity in Gpr54> −/− -Tg rescue mice. Mean+s.e.m. values showing ( a ) the day of vaginal opening in three genotypes ( n =6 each). ( b ) Estrous cycle length in three genotypes ( n =6 each); wild-type and Gpr54 −/− ;Tg rescue are not significantly different. ( c ) Fecundity over 120 days for three representative individual female mice (each line) from each genotype with symbols showing the times at which each litter was born. Gpr54 −/− mice failed to generate any litters. ( d ) Onset of reproductive competence for male mice of three genotypes ( n =6 each). Gpr54 −/− mice failed to sire any litters. ( e ) Pups per litter were not different between wild-type and Gpr54 −/− ;Tg rescue male mice. ( f ) Fecundity over 120 days for three representative individual male mice (each line) from each genotype. Full size image The fertility of Gpr54 −/− females was also rescued by the Gpr54 −/− ;Tg transgene. The sizes of the uterus and ovary of wild-type and Gpr54 −/− ;Tg mice were not different with normally developed ovaries and uteri, whereas those of Gpr54 −/− mice were markedly reduced ( Fig. 4c ). Whereas vaginal opening was absent in Gpr54 −/− mice, the Gpr54 −/− ;Tg rescue animals exhibited vaginal opening at the same time as wild-type mice ( n =6, each genotype; Fig. 9a ). Subsequent vaginal smearing of these mice as adults showed a return of estrous cycles to Gpr54 −/− ;Tg rescue mice with a length (5.2±0.2 days (s.e.m.)) similar to that of wild-type mice (6.3±0.5). Gpr54 −/− continued to show an absence of vaginal opening ( Fig. 9b ). In 4-month mating trials, Gpr54 −/− ;Tg rescue ( n =6) and wild-type animals ( n =6) produced similar numbers of litters (5.0±0.6 (s.e.m.) versus 3.8±1.1) and pups per litter (8.6±0.7 versus 7.1±1.1) ( Fig. 9c ). Basal LH levels were not significantly different among the three genotypes in either sex ( Fig. 10 ), although FSH levels were markedly reduced in global Gpr54 −/− male ( P <0.001; ANOVA, post hoc Tukey test) and female ( P <0.05) mice compared with wild-type mice, and these values were returned to normal levels in Gpr54 −/− ;Tg mice ( P <0.001 both sexes; Fig. 10 ). 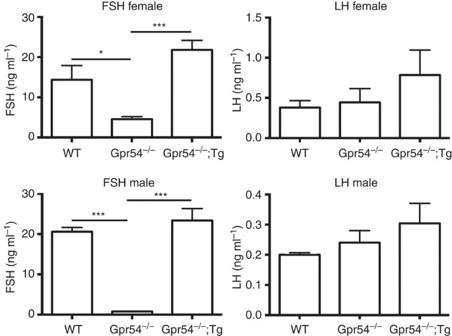Figure 10: Basal FSH and LH levels in rescue mice. Mean+s.e.m. values are given for wild-type (WT), Gpr54 knockout (Gpr54−/−) and Gpr54 knockout; transgene rescue (Gpr54−/−;Tg) adult male and female mice. (n=5 per group). FSH female, ANOVAP=0.001, *P<0.05, ***P<0.001. FSH male, ANOVAP=0.001, ***P<0.001. LH male and female, ANOVAP>0.05. Figure 10: Basal FSH and LH levels in rescue mice. Mean+s.e.m. values are given for wild-type (WT), Gpr54 knockout (Gpr54 −/− ) and Gpr54 knockout; transgene rescue (Gpr54 −/− ;Tg) adult male and female mice. ( n =5 per group). FSH female, ANOVA P =0.001, * P <0.05, *** P <0.001. FSH male, ANOVA P =0.001, *** P <0.001. LH male and female, ANOVA P >0.05. Full size image We report here that the deletion of Gpr54 from GnRH neurons results in infertility, whereas the re-introduction of Gpr54 to GnRH neurons in global Gpr54 mutant mice rescues fertility. These reciprocal phenotypes indicate that Gpr54 signaling at the GnRH neuron is both essential and sufficient for reproduction in mice. These studies rely on GnRH BAC transgenesis to target the expression of GFP, Cre and Gpr54 to GnRH neurons in a selective manner. Accordingly, we have undertaken a range of immunohistochemical, electrophysiological and tissue-profiling characterization studies in these mouse lines. These have found evidence for highly efficient (~98%) and consistent targeting of the GnRH neuronal phenotype in a selective manner. This is in good agreement with other studies using the same mice [25] , [26] and GnRH transgenics using short promoters [32] , [33] . We note, however, that this strategy also targets cells in the LSi and in some instances the BNST, where GnRH transgenes unavoidably drive expression [28] . This is unlikely to represent any major confound for the present investigations, as Gpr54 is not expressed in the BNST and has been identified in only a very few cells in the intermediate division of the LS [18] . The four eGFP and five Tg mouse lines were all generated with the same GnRH BAC transgene and provided identical targeting and phenotypes. This indicates that the 200-kb BAC used in these studies provides good insulation from flanking DNA sequences following insertion into the genome, as well as the regulatory elements required for targeting GnRH neurons. Whereas it is likely that GnRH is expressed in other tissues, such as the gonads [34] , [35] , it appears that the GnRH transgenics used here do not drive sufficient transgene expression for detection, or in the case of Cre, functional recombination. By developing an assay of kisspeptin action on ERK1/2 and Akt phosphorylation in the pituitary gland, we were also able to provide functional evidence that the pituitary gland is not targeted in Gpr54 −/− ;Tg rescue mice. We note that the effects of kisspeptin on these signaling cascades appear to be quite cell-specific as, for example, kisspeptin suppresses Akt phosphorylation but stimulates ERK1/2 phosphorylation in cancer cell lines [31] . The results of the electrophysiological analysis confirmed the deletion or re-introduction of functional Gpr54 in GnRH neurons in the mutant mouse models. Whereas the kisspeptin responses of GnRH neurons in control lines were normal, occurring in ~65–80% of the population, not a single GnRH neuron responded to kisspeptin in global Gpr54 −/− or GnRH neuron-targeted Gpr54 −/− mice. In contrast, the transgene-rescue strategy returned kisspeptin responsiveness to nearly 70% of GnRH neurons. Intriguingly, we noted that the basal firing rates of GnRH neurons appeared to be dependent on their Gpr54 status. Normal or control GnRH neurons exhibited mean firing rates of 0.8 Hz, whereas those without Gpr54 in global or GnRH neuron-selective Gpr54 knockouts exhibited very low firing in the range of 0.07–0.16 Hz. This suggests the potential importance of kisspeptin–Gpr54 signaling in enabling GnRH neurons to maintain a normal level of excitability while also showing that some GnRH neuron activity remains in the absence of Gpr54 (ref. 36 ). Unexpectedly, GnRH neurons in rescue mice were found to exhibit a very high basal firing rate. The reasons for this are not clear, although altered amino-acid transmission can be ruled out, and it may represent upregulated expression of Gpr54 in GnRH neurons as it is now driven by the GnRH promoter. Against this possibility, however, we note that the response of GnRH neurons to exogenous kisspeptin in Gpr54 knockin mice was similar to that of GnRH neurons in normal GnRH-GFP animals. Intriguingly, despite exhibiting a much higher basal GnRH neuron-firing rate, at least in the acute brain-slice preparation, the reproductive axis of rescue mice in vivo , including their gonadotropin levels, appears normal in all respects. Mayer and Boehm [19] reported that diphtheria toxin ablation of most kisspeptin-expressing neurons during embryogenesis does not influence substantially their later reproductive capacity, although postnatal deletion of kisspeptin neurons results in infertility. This is in contrast to genetic mutations of Kiss1 or Gpr54 that are uniformly infertile [1] , [36] , [37] . The reasons for the different fertility phenotypes resulting from prenatal genetic deletion of Kiss1 and prenatal toxin ablation of kisspeptin neurons are not understood. One possibility is that the deletion of kisspeptin neurons provides a greater stimulus for compensation and re-wiring in the developing brain compared with deletion of just the peptide. Another plausible explanation is that there may be sufficient redundancy in the kisspeptin neuron populations such that even a 95% reduction in kisspeptin number following toxin ablation is compatible with at least some degree of fertility [38] . With GnRH1 being expressed from mid-gestation onwards in the mouse, the GnRH neuron-specific knockin and knockout of Gpr54 reported here will have been in place well before birth, simulating the genetic defects of the global Kiss1 or Gpr54 null lines. As such, it is not surprising to find that GnRH-Cre +/− ;Gpr54 f/f mice replicate the phenotype of global Gpr54 mutants that are invariably anovulatory and infertile with reduced gonadal size and FSH levels (for review see Colledge [39] ). Of note, however, one Gpr54 mutant line is reported to be infertile but nevertheless transitions to estrous at ~9 months of age [36] , beyond the 6-month period of analysis used in the present study. Approximately 20% of GnRH neurons do not express Gpr54 (refs 17 , 18 ) and would be assumed to be unaffected in global or, as here, GnRH neuron-specific deletions of Gpr54. Given that relatively few GnRH neurons (10–30%) are actually required for normal fertility in mice [19] , [40] , [41] , it is curious that these Gpr54-lacking GnRH neurons are insufficient for reproductive competence. However, as only 50–70% of all GnRH neurons are thought to be involved in controling pituitary gonadotropin secretion [42] , [43] , it is possible that the 20% of GnRH neurons that do not express Gpr54 are involved in other functions of GnRH within the brain. Increasing evidence has been found for roles of kisspeptin and Gpr54 in a variety of reproductive tissues [8] , [9] , [10] , [11] , [12] , [13] . The full recovery of reproductive function in Gpr54 −/− ;Tg rescue mice indicates that kisspeptin–Gpr54 signaling at other sites in the HPG axis, and the placenta, is not essential for reproduction. It seems likely that the effects of kisspeptin and Gpr54 activation in these tissues serve modulatory purposes or, at least, can be compensated for in terms of reproductive efficiency. In contrast, the present observations indicate that kisspeptin–Gpr54 signaling at the GnRH neuron is essential in mice and likely represents the key locus for kisspeptin control of fertility in all mammals. Generation of mice All experimentation was approved by the University of Otago Animal Welfare and Ethics Committee with mice maintained under 12-h light, 12-h dark lighting conditions, with food and water ad libitum . New mouse lines were backcrossed to the C57BL/6 background. A standard cloning strategy was used to flox exon two of Gpr54 ( Fig. 1a ). The deletion of exon two will lead to a frameshift and nonfunctional protein. The targeting vector was constructed by cloning a 2.5-kb 5′ homology arm upstream of the LoxP-Frt-tkneo-Frt fusion cassette in Bluescript KS+ vector using Not I and Pml I restriction enzymes. The 3′ homology arm was introduced in two steps. In the first step, a PCR fragment containing exon two and the second LoxP element was cloned downstream of the tkneo cassette by Pac I and Ssp I. In the second step, a homology arm with size of 3.8 kb was cloned downstream of the LoxP element by Sna BI and Asc I. The final targeting vector was linearized by Hpa I and electroporated in mouse ES cells. The screening of the ES clones for the right integration was performed using Southern blot with external of the homology arm probes. Mice were genotyped using the following primers; Pr.7841_F, 5′-CCTGTTTTTCGCTACACTCATGTTGCTTGGTG-3′; Pr.8348_R, 5′-AGAGAAACTTAGGCTCCCCCACCCTCCTT-3′; Pr.9375_R, 5′-GACTCTCCCTTAAGCCCTACCCCACACATC-3′; resulting in a 507-bp band for wild types, a 593-bp band for the floxed allele and a 836-bp band following recombination. BAC recombineering was used to generate transgenic mice targeting either Gpr54- or GFP-coding sequences to GnRH neurons. In brief, targeting vectors with Gpr54 or GFP cDNAs with two short homology arms of 50 bp were recombined in an ~200-kb GnRH BAC (RP23-358B23), replacing a sequence in the first exon of the GnRH1 gene ( Fig. 4a ). Mice were genotyped using the following primer sets: T1003E, 5′-GCCTAAGTTTCTCTGGTGGAGGATG-3′; T1003TE, 5′-CGCGTACCTGCTGGATGTAGTTGAC-3′; NeoT, 5′-GGGTGGGATTAGATAAATGCCTGCTCT-3′, resulting in a wt band of 253 bp and a knockout band of 455 bp. A separate PCR was performed to show the presence of the rescue transgene (439 bp) using primers GnRH_F, 5′-GGTTTCAGGGAACCCAAATTA-3′ and GPR54_R, 5′-ACCAATGAGTTTCCGACCAG-3′. Histochemistry GnRH immunohistochemistry combined with Xgal histochemistry was undertaken as reported previously [18] . This involved anesthetizing adult (~90 days of age) female GnRH-Cre +/− ; ROSA26::LoxP-Stop-LoxP-LacZ mice with Pentobarbital, followed by perfusion through the heart with a 4% paraformaldehyde solution. Brains were removed and cut into 30 μm-thick coronal slices through the rostral hypothalamus and placed overnight in 2% Xgal to generate a blue reaction product. The sections were then washed and placed in a polyclonal rabbit GnRH antisera (LR1 at 1:40,000; gift of R. Beniot, Montreal) for 48 h at 4 °C before being washed and placed in biotinylated goat anti-rabbit immunoglobulins (1:400; Vector Labs) for 90 min at room temperature (RT) followed by Vector Elite avidin-peroxidase (1:100; Vector Labs) for 90 min at RT. GnRH immunoreactivity was revealed using glucose oxidase-reacted diaminobenzidine hydrochloride (DAB). Cre immunohistochemistry was undertaken on 18-μm-thick coronal sections of 4% paraformaldehyde perfusion-fixed brain, pituitary, ovary and testis obtained from adult (>90 days of age) male and female GnRH-Cre mice. Single-label slide-mounted immunohistochemistry was conducted using a well-characterized antisera raised against Cre (1:10,000; G. Schütz, Heidelberg) [44] with nickel-DAB as chromagen. Dual-labelling GnRH-Cre immunohistochemistry was undertaken using a previously reported protocol [26] in which free-floating 30-μm-thick sections from GnRH-Cre mice were first stained for Cre with nickel-DAB as chromagen (as above) and then treated with 30% ethanol and 2% hydrogen peroxide to destroy any remaining peroxidase activity and put through the LR1 GnRH immunohistochemistry procedure (as above) using DAB alone used as the chromagen for revealing GnRH immunoreactivity. GFP immunohistochemistry was undertaken on coronal sections of 4% paraformaldehyde perfusion-fixed brain, pituitary, ovary and testis obtained from adult (~90 days of age) male and female GnRH-GFP mice. Single-label slide-mounted immunohistochemistry was conducted using a rabbit polyclonal antisera raised against GFP (1:5,000, Molecular Probes) [45] for 48 h at 4 °C, with nickel-DAB as chromagen. Electrophysiology Cell-attached recordings were made from adult female (65–120 days old) C57BL/6 GFP-tagged GnRH neurons in the coronal brain-slice preparation as described previously [24] , [46] . In brief, following decapitation and quick removal of the brain, 250-μm-thick coronal brain slices containing rostral preoptic area were prepared with a vibratome and placed in the recording bath of a fixed-stage upright microscope (BX51WI; Olympus, Tokyo) receiving equilibrated (95% O 2 , 5% CO 2 ) artificial cerebrospinal fluid containing (in mM) 118 NaCl, 3 KCl, 2.5 CaCl 2 , 1.2 MgCl 2 , 11 D-glucose, 10 HEPES and 25 NaHCO 3 at 2-3 ml min −1 and maintained at 32±1 °C. GnRH neurons in the various GnRH-GFP lines were identified by the presence of GFP, revealed by brief illumination with blue light, and then patched under differential interference contrast optics. Patch pipettes had 3–5 M Ohm resistances when filled with the pipette solution composed of (in mM) 145 NaCl, 3 KCl, 2.5 CaCl 2 , 10 HEPES, 1.2 MgCl 2 (pH 7.4 adjusted with NaOH, ~290 mOs mol). Signals were acquired using a Multiclamp 700B amplifier (Molecular Devices, Sunnyvale, CA) connected to a Digidata 1440A (Axon Instruments, Union City, CA) and low-pass filtered at 10 kHz before being digitized at 10 kHz. Acquisition and subsequent analysis of the acquired data were performed with the Clampex 10 suite of software (Molecular Devices) and Origin Pro 7.5 (OriginLab Corporation, Northampton, MA, USA). Kisspeptin (100 nM) was bath-applied in the presence or absence of an ionotropic glutamate and GABA A receptor antagonist cocktail including 2 mM kynurenic acid, 20 μM CNQX and 5 μM gabazine (AAB). In vitro pituitary studies To ensure equal circulating estradiol concentrations among the three adult female genotypes (wild type, Gpr54 −/− , rescue Gpr54 −/− ;Tg; n =8 each, ~90 days old), mice were implanted with Silastic capsules (10 mm length; inner diameter, 0.062 cm) containing 17-β-estradiol (100 μg ml −1 ). Two weeks later, pituitary tissue was processed as described previously [47] . Briefly, entire pituitary glands were quickly removed and incubated in 2 ml Dulbecco's Modified Eagle Medium on a shaker at 37 °C at 95% O 2 and 5% CO 2 . After 45-min pre-incubation, the media were replaced either by fresh media or by one containing 10 nM kisspeptin. Pituitary glands were collected after 10 min, frozen in liquid nitrogen and stored at –80 °C. Total protein lysates (10 μg) were then subjected to SDS–PAGE electrophoresis and transferred on polyvinyl difluoride membranes. Membranes were probed for 16 h at 4 °C in the presence of antibodies directed against phosphorylated (p)-AKT (1:2,000, Cell Signaling, Danvers, MA), pERK1/2 (1:2,000; Cell Signaling) and α-Tubulin (1:10,000; Sigma-Aldrich). Protein detection was performed using horseradish peroxidase-conjugated secondary antibodies and enhanced chemiluminescence reagent (Amersham, Aylesbury, UK). Reproductive profiling Assessments of puberty onset, estrous cyclicity and fecundity were performed as reported previously [40] . For females, this involved examining for the day of vaginal opening from postnatal day 25 onwards and by subsequent daily vaginal smear cytology to determine the day of first estrous. Further daily vaginal smearing from postnatal day 60 onwards for a period of 2 weeks was used to assess estrous cyclicity. Mating performance was assessed by placing a mutant or control female (> postnatal day 60) with an adult wild-type stud male and counting the numbers of litters and pups per litter produced over the following 4 months. For male mice, an adult (> postnatal day 60) wild-type female mouse was placed with the mutant male from day 35 onwards and the time of birth of the first litter was used to back-calculate the first day of successful mating for the male mouse (time of first litter born minus 20 days). Mating performance was undertaken by placing mutant or control males at >60 day of age with wild-type female mice and the numbers of litters and pups per litter counted over the following 4 months. The in vivo kisspeptin challenge was adapted from D’Anglemont de Tassigny et al. [48] and involved administering a single intraperitoneal injection of 100 μl of 1 mM kisspeptin in saline or 100 μl of saline (vehicle control) to adult male (60–90 days) mice of each genotype (GnRH-Cre +/− ;Gpr54 f/f or Gpr54 f/f ). Mice were killed by decapitation 10 min after injection and blood was collected from the trunk into a heparinized tube. Plasma was separated by centrifugation at 4,000 g for 10 min and then stored at −20 °C until assayed. LH levels were determined using radioimmunoassay (RIA) as reported previously [40] . Basal FSH levels were assessed by RIA using the anti-mFSH and mFSH-RP reference provided by Dr A.F. Parlow (National Hormone and Pituitary Program, Torrance, CA). The RIA intra-assay coefficients of variation were 8.9% for LH and 0.7% for FSH. The inter-assay coefficient of variation for LH was 10.3%. Statistical analysis was undertaken by non-parametric Mann–Whitney U -test for experimental groups of two and by ANOVA with Tukey post hoc tests for groups larger than two unless stated otherwise. How to cite this article: Kirilov, M. et al. Dependence of fertility on kisspeptin–Gpr54 signaling at the GnRH neuron. Nat. Commun. 4:2492 doi: 10.1038/ncomms3492 (2013).